Proinflammatory TLR signalling is regulated by a TRAF2-dependent proteolysis mechanism in macrophages Signal transduction from toll-like receptors (TLRs) is important for innate immunity against infections, but deregulated TLR signalling contributes to inflammatory disorders. Here we show that myeloid cell-specific ablation of TRAF2 greatly promotes TLR-stimulated proinflammatory cytokine expression in macrophages and exacerbates colitis in an animal model of inflammatory bowel disease. TRAF2 deficiency does not enhance upstream signalling events, but it causes accumulation of two transcription factors, c-Rel and IRF5, known to mediate proinflammatory cytokine induction. Interestingly, TRAF2 controls the fate of c-Rel and IRF5 via a proteasome-dependent mechanism that also requires TRAF3 and the E3 ubiquitin ligase cIAP. We further show that TRAF2 also regulates inflammatory cytokine production in tumour-associated macrophages and facilitates tumour growth. These findings demonstrate an unexpected anti-inflammatory function of TRAF2 and suggest a proteasome-dependent mechanism that limits the proinflammatory TLR signalling. Macrophages form a major type of innate immune cells that mediate host defense against infections and inflammatory responses [1] . On activation, macrophages produce various proinflammatory cytokines and other factors that regulate inflammation and the early phase of an immune response. The activation and function of macrophages rely on innate immune receptors, particularly the pattern-recognition receptors (PRRs) that detect various molecular patterns associated with the invading pathogens [2] . One major family of PRRs is the toll-like receptors (TLRs), which function on the cell surface or intracellular compartments [3] . Stimulation of the TLRs by specific ligands initiates cascades of signalling events through MyD88- and TRIF-dependent pathways, leading to the activation of three major families of MAP kinases (MAPKs), ERK, JNK and p38, as well as the IκB kinase (IKK). The MAPKs mediate activation of the transcription factors AP-1 and CEBPs, and the IKK engages in activation of the transcription factor NF-κB (ref. 2 ). The NF-κB family of transcription factors plays a crucial role in transactivating genes encoding proinflammatory cytokines [4] , [5] . In particular, the NF-κB member c-Rel is specifically required for TLR-stimulated expression of IL-12 and IL-23 (refs 6 , 7 , 8 ). Besides the traditional transcription factors, interferon-responsive factor 5 (IRF5) is required for TLR-stimulated proinflammatory cytokine induction [9] , [10] . IRF5 mediates induction of multiple proinflammatory cytokines, such as IL-6, IL-12, IL-23, and tumour-necrosis factor-alpha (TNF-α), and inhibits induction of the anti-inflammatory cytokine IL-10 (refs 9 , 10 ). Both IRF5 and c-Rel have been associated with human inflammatory diseases [11] , [12] , [13] , [14] , but how these proinflammatory mediators are negatively regulated during the macrophage differentiation and activation remains unknown. TNFR-associated factors (TRAFs) are important mediators of innate immune receptor signalling [15] . TRAF6 is essential for TLR-stimulated activation of MAPKs and IKK and induction of proinflammatory cytokines [16] , but the role of the other TRAF family members in regulating TLR signalling is less clear. TRAF2 is known as an adaptor involved in activation of MAPKs and IKK by TNF receptors (TNFRs), such as TNFR1 and CD40 (refs 17 , 18 ). However, the role of TRAF2 in regulating TLR signalling in innate immune cells and inflammation has been elusive. Notably, elevated expression of TRAF2, as well as its homologue TRAF3, is associated with human inflammatory bowel disease (IBD) [19] , [20] , [21] . Higher TRAF2 expression is also a predictor of relapse in patients with ulcerative colitis (UC) [20] , although how TRAF2 regulates colon inflammation is unclear. In the present study, we addressed this question by generating myeloid cell-conditional knockout mice. We found that myeloid cell-specific ablation of TRAF2 greatly promotes TLR-stimulated proinflammatory cytokine expression in macrophages and exacerbates colitis in an animal model of IBD. We obtained genetic and biochemical evidence that TRAF2 mediates proteasome-dependent degradation of the proinflammatory transcription factors IRF5 and c-Rel in a mechanism that also requires TRAF3 and the E3 ubiquitin ligase cIAP (cIAP1 or cIAP2). We further show that TRAF2 regulates macrophage polarization in tumour microenvironment and plays a role in controlling tumour growth. These findings reveal an unexpected anti-inflammatory function of TRAF2 in macrophages and highlight a novel mechanism that limits the proinflammatory TLR signalling. Myeloid cell-specific TRAF2 ablation promotes colitis TRAF2 overexpression is associated with human IBD and IBD recurrence, although it has remained unclear whether TRAF2 plays a role in innate immune cells to promote or inhibit colon inflammation [19] , [20] , [21] . To address this question, we employed a widely used animal model of IBD, the dextran sodium sulfate (DSS)-induced colitis [22] . Interestingly, the level of TRAF2, as well as its homologue TRAF3, was substantially higher in the colonic macrophages, compared with that in splenic and peritoneal macrophages ( Fig. 1a ). As this result was seen in both untreated and DSS-treated mice, the higher level of TRAF2 and TRAF3 might be due to the homeostatic conditions of the colon, in which immune cells have a dynamic interaction with commensal microbes. To examine the function of TRAF2 in regulating colon inflammation, we generated myeloid cell-conditional TRAF2-knockout ( Traf2 -MKO) mice by crossing the Traf2 -flox mice with Lyz2 -Cre mice. The Traf2 -MKO mice did not show appreciable changes in the frequency of macrophages or neutrophils ( Supplementary Fig. 1a ). 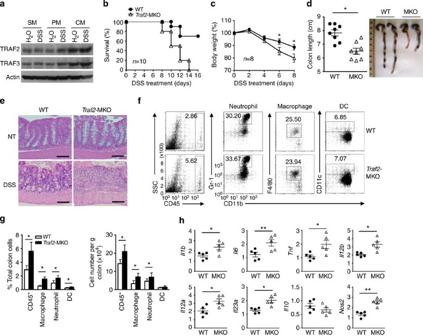Figure 1: TRAF2 negatively regulates experimental colitis. WT andTraf2-MKO (T2-MKO) mice were treated with 3% (a,c–h) or 3.5% (b) DSS (in drinking water) for 6 days and then supplied with normal drinking water. (a) IB analysis of TRAF2 and TRAF3 in the FACS-sorted spleen (SM), peritoneal (PM) and colon (CM) macrophages (CD11b+F4/80+) from naive (H2O treated) and day 8 DSS-treated WT mice. (b,c) Survival rate (b) and body weight loss (c) of DSS-treatedTraf2-MKO and WT mice. (d,e) Colon Length (d) and H&E histology staining (e) from day 8 DSS-treatedTraf2-MKO and WT mice. (Scale bar, 100 μm) (f,g) FACS analysis of the total immune cells (CD45+) and the indicated subsets, presented as a representative plot (f) and mean±s.d. values of multiple mice (n=3 mice/genotype) (g). (h) qRT-PCR analysis of the indicated genes (presented as fold relative toActinmRNA level) using FACS-sorted colon macrophages (CD11b+F4/80+) from day 8 DSS-treated WT andTraf2-MKO mice. Data shown are representative of at least three independent experiments. The error bars represent standard deviation (s.d.). Differences between experimental and control groups were determined by Student’st-test. For animal survival analysis, the Kaplan–Meier method was adopted to generate graphs, and the survival curves were analysed with log-rank analysis. *P<0.05; **P<0.01. Figure 1: TRAF2 negatively regulates experimental colitis. WT and Traf2 -MKO (T2-MKO) mice were treated with 3% ( a , c – h ) or 3.5% ( b ) DSS (in drinking water) for 6 days and then supplied with normal drinking water. ( a ) IB analysis of TRAF2 and TRAF3 in the FACS-sorted spleen (SM), peritoneal (PM) and colon (CM) macrophages (CD11b + F4/80 + ) from naive (H 2 O treated) and day 8 DSS-treated WT mice. ( b , c ) Survival rate ( b ) and body weight loss ( c ) of DSS-treated Traf2 -MKO and WT mice. ( d , e ) Colon Length ( d ) and H&E histology staining ( e ) from day 8 DSS-treated Traf2 -MKO and WT mice. (Scale bar, 100 μm) ( f , g ) FACS analysis of the total immune cells (CD45 + ) and the indicated subsets, presented as a representative plot ( f ) and mean±s.d. values of multiple mice ( n =3 mice/genotype) ( g ). ( h ) qRT-PCR analysis of the indicated genes (presented as fold relative to Actin mRNA level) using FACS-sorted colon macrophages (CD11b + F4/80 + ) from day 8 DSS-treated WT and Traf2 -MKO mice. Data shown are representative of at least three independent experiments. The error bars represent standard deviation (s.d.). Differences between experimental and control groups were determined by Student’s t -test. For animal survival analysis, the Kaplan–Meier method was adopted to generate graphs, and the survival curves were analysed with log-rank analysis. * P <0.05; ** P <0.01. Full size image We then examined the myeloid cell-specific role of TRAF2 in the regulation of colon inflammation using the DSS-induced colitis model. When fed with drinking water containing 3.5% DSS, as high as 70% of the wild-type (WT) mice survived the treatment up to 16 days ( Fig. 1b ). In sharp contrast, 100% of the Traf2 -MKO mice died within 14 days of DSS treatment ( Fig. 1b ). For studying the phenotypes of colon inflammation, we treated the mice with a lower dose of DSS to prevent early death. Compared with the WT mice, the Traf2 -MKO mice had significantly reduced bodyweight and shortened the colon, typical features of colitis ( Fig. 1c,d ). Consistently, histology analyses revealed exacerbated inflammation in the distal colon of the TRAF2-deficient mice, characterized by enhanced leukocyte infiltration and more severe mucosal damage ( Fig. 1e ). Flow cytometry also detected increased frequency and number of colon-infiltrating immune cells (CD45 + ) ( Fig. 1f,g ). Although the gated CD45 + cells of WT and Traf2 -MKO mice did not differ substantially in the frequency of myeloid cell subsets ( Fig. 1f ), the frequency of these cells within the total colon cells was significantly increased in the Traf2 -MKO colon due to the substantial elevation in the total population of the infiltrating CD45 + immune cells ( Fig. 1g , left panel). The absolute number of macrophages and neutrophils was also significantly elevated in the Traf2 -MKO colon ( Fig. 1g , right panel). Furthermore, real-time quantitative RT-PCR (qRT-PCR) assays revealed elevated expression of a number of proinflammatory cytokine genes in the colonic macrophages of the Traf2 -MKO mice ( Fig. 1h ). In contrast, the loss of TRAF2 caused a moderate reduction in the expression of the anti-inflammatory cytokine gene Il10 ( Fig. 1h ). These results establish TRAF2 as a negative regulator of colitis that functions in innate immune cells. TRAF2 inhibits proinflammatory cytokine induction To examine the mechanism by which TRAF2 regulates colitis, we analysed the effect of TRAF2 deficiency on gene induction in macrophages by the TLR4 ligand LPS. Remarkably, the TRAF2-deficient bone marrow-derived macrophages (BMDMs) were hyper-responsive to LPS in the induction of a number of proinflammatory cytokine genes and the iNOS gene ( Nos2 ) ( Fig. 2a ). Conversely, the TRAF2 deficiency attenuated the induction of the anti-inflammatory cytokine gene Il10 . Similar results were obtained using peritoneal macrophages isolated from the Traf2 -MKO or WT control mice ( Fig. 2b ). The LPS-stimulated aberrant expression of proinflammatory cytokines in Traf2 -MKO macrophages also occurred at the protein level, as revealed by ELISA ( Fig. 2c ). 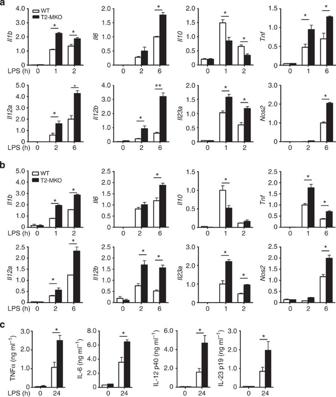Figure 2: TRAF2 negatively regulates proinflammatory cytokine induction. (a,b) qRT-PCR analysis of the indicated genes using BMDMs (a) or peritoneal macrophages (b) derived from WT orTraf2-MKO mice at 0, 2 and 6 h after LPS stimulation. Data are presented as fold relative to theActinmRNA level. (c) ELISA of the indicated cytokines in the supernatants of the WT andTraf2-MKO BMDMs, which were either not treated (0) or stimulated with LPS for 24 h. Data are presented as mean±s.e.m. values and representative of at least three independent experiments. The error bars represent s.d., and differences between experimental and control groups were determined by Student’sttest. *P<0.05; **P<0.01. Figure 2: TRAF2 negatively regulates proinflammatory cytokine induction. ( a , b ) qRT-PCR analysis of the indicated genes using BMDMs ( a ) or peritoneal macrophages ( b ) derived from WT or Traf2 -MKO mice at 0, 2 and 6 h after LPS stimulation. Data are presented as fold relative to the Actin mRNA level. ( c ) ELISA of the indicated cytokines in the supernatants of the WT and Traf2 -MKO BMDMs, which were either not treated (0) or stimulated with LPS for 24 h. Data are presented as mean±s.e.m. values and representative of at least three independent experiments. The error bars represent s.d., and differences between experimental and control groups were determined by Student’s t test. * P <0.05; ** P <0.01. Full size image To examine whether TRAF2 also regulates gene induction by other immune stimuli, we stimulated the WT and TRAF2-deficient BMDMs and peritoneal macrophages with the TLR3 agonist poly(I:C). Like LPS, poly(I:C) stimulated hyper-expression of several proinflammatory cytokine genes and reduced expression of Il10 in the TRAF2-deficient BMDMs and peritoneal macrophages ( Supplementary Fig. 1b,c ). Similar results were also obtained when the macrophages were stimulated with IL-1β, which is known to induce signalling via the MyD88 pathway ( Supplementary Fig. 1d ). Collectively, these results demonstrated an unexpected anti-inflammatory function of TRAF2 in the TLR pathway, providing mechanistic insight into the colitis-regulatory role of TRAF2. Antiinflammatory function of TRAF2 is independent of NIK TRAF2 is known as a negative regulator of the noncanonical NF-κB pathway [23] , [24] . Indeed, the TRAF2 deficiency in macrophages caused accumulation of NIK and concomitant processing of p100 to generate p52 ( Fig. 3a ). Furthermore, as previously reported [25] the NIK accumulation also enhanced some of the canonical NF-κB signalling events, including phosphorylation of the NF-κB inhibitor IκBα and the canonical NF-κB member p65 at serine 529 ( Fig. 3a ). These signalling events were largely, although not completely, dependent on NIK, as they were diminished in NIK-null genetic background ( Fig. 3a ). It is currently unclear how the loss of TRAF2 caused the residual basal level phosphorylation of IκBα and p65 in the NIK-deficient background. Similar results were obtained with the Traf3 -MKO macrophages (data not shown). 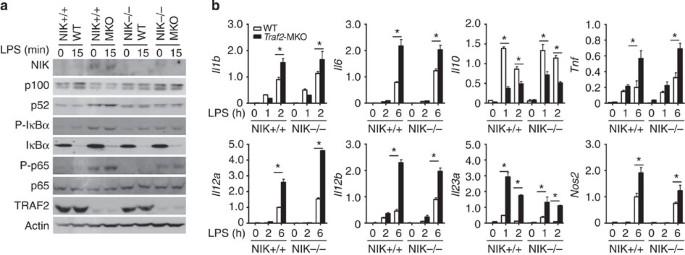Figure 3: TRAF2 negatively regulates proinflammatory cytokine induction independently of NIK. (a) IB analysis of the indicated phosphorylated (P-) and total proteins in the whole-cell lysates of LPS-stimulated BMDMs derived from WT orTraf2-MKO (MKO) mice crossed to NIK+/+or NIK−/−background. (b) qRT-PCR analysis of the indicated mRNAs in LPS-stimulated BMDMs derived from the WT andTraf2-MKO mice crossed to NIK+/+or NIK−/−background. The mRNA level was calculated as fold relative to an internal control,Actb. Data are mean±s.e.m. based on multiple samples and representative of three independent experiments. The error bars represent s.d., and differences between experimental and control groups were determined by Student’st-test. *P<0.05. Figure 3: TRAF2 negatively regulates proinflammatory cytokine induction independently of NIK. ( a ) IB analysis of the indicated phosphorylated (P-) and total proteins in the whole-cell lysates of LPS-stimulated BMDMs derived from WT or Traf2 -MKO (MKO) mice crossed to NIK +/+ or NIK −/− background. ( b ) qRT-PCR analysis of the indicated mRNAs in LPS-stimulated BMDMs derived from the WT and Traf2 -MKO mice crossed to NIK +/+ or NIK −/− background. The mRNA level was calculated as fold relative to an internal control, Actb . Data are mean±s.e.m. based on multiple samples and representative of three independent experiments. The error bars represent s.d., and differences between experimental and control groups were determined by Student’s t -test. * P <0.05. Full size image To examine the functional significance of noncanonical NF-κB activation in the induction of proinflammatory cytokine genes, we prepared BMDMs from WT and Traf2 -MKO mice, either in NIK +/+ or NIK −/− (NIK-KO) background. As expected, the TRAF2 deficiency in NIK +/+ background caused hyper-induction of several proinflammatory cytokine genes and downregulation of the anti-inflammatory Il10 gene ( Fig. 3b ). Importantly, such an abnormal gene induction phenotype was not corrected on ablation of NIK, with the exception of Il23a that was partially downregulated in the NIK-null background ( Fig. 3b ). These results suggest that the noncanonical NF-κB pathway does not play a major role in the regulation of TLR-stimulated proinflammatory gene induction in macrophages. TRAF2 mediates degradation of c-Rel and IRF5 Induction of proinflammatory cytokines by LPS involves activation of the MAP kinase kinase kinase (MAP3K) TAK1 and its downstream IKK and MAPKs (p38 and JNK). The TRAF2 deficiency did not promote, but rather moderately inhibited, LPS-stimulated activation of the typical IKK complex, as revealed by an in vitro kinase assay ( Fig. 4a ). This result was somewhat surprising, as the TRAF2-deficient macrophages had higher basal level phosphorylation of IκBα and p65 ( Fig. 3a ). Although precisely how TRAF2 deficiency enhanced basal level of IκBα/p65 phosphorylation is unclear, it appeared that this is at least partially mediated by the NIK pathway, as these phosphorylation events were substantially, although not completely, inhibited on NIK ablation ( Fig. 3a ). We also found that LPS-stimulated activation of TAK1 and its targets p38 and JNK was comparable between the WT and Traf2 -MKO macrophages ( Fig. 4b ). 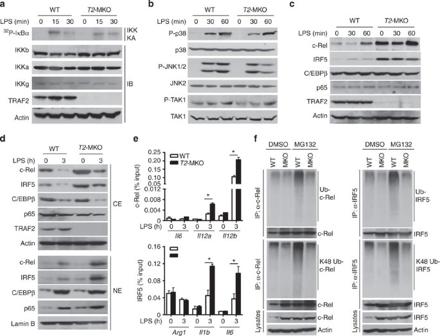Figure 4: TRAF2 deficiency attenuates ubiquitin-dependent degradation of c-Rel and IRF5 and promotes their function. (a) IKK kinase assay (KA) and IB assays using whole-cell lysates of LPS-stimulated BMDMs derived from WT andTraf2-MKO mice. (b,c) IB analysis of the indicated phosphorylated (P-) and total proteins in whole-cell lysates of WT andTraf2-MKO BMDMs stimulated with LPS. (d) Immunoblot analysis of the indicated proteins in the cytoplasmic (CE) and nuclear (NE) extracts of WT andTraf2-MKO BMDMs either not treated (0) or stimulated with LPS for 3 h. (e) ChIP analysis of c-Rel and IRF5 at the promoter of the indicated genes using WT orTraf2-MKO BMDMs that were either not treated (0) or stimulated for 3 h with LPS. Data are presented as fold relative to the total input DNA and representative of three or more independent experiments. *P<0.05. (f) IRF5 and c-Rel were isolated by IP (under denaturing conditions) from whole-cell lysates of DMSO or MG132-treated WT andTraf2-MKO BMDMs and subjected to IB assays using anti-ubiquitin (top panels) or anti-K48-linked ubiquitin (middle panels) antibodies. Protein lysates were also subjected to direct IB (bottom panels). Data are representative of at least three independent experiments. The error bars represent s.d., and differences between experimental and control groups were determined by Student’st-test. *P<0.05. Figure 4: TRAF2 deficiency attenuates ubiquitin-dependent degradation of c-Rel and IRF5 and promotes their function. ( a ) IKK kinase assay (KA) and IB assays using whole-cell lysates of LPS-stimulated BMDMs derived from WT and Traf2 -MKO mice. ( b , c ) IB analysis of the indicated phosphorylated (P-) and total proteins in whole-cell lysates of WT and Traf2 -MKO BMDMs stimulated with LPS. ( d ) Immunoblot analysis of the indicated proteins in the cytoplasmic (CE) and nuclear (NE) extracts of WT and Traf2 -MKO BMDMs either not treated (0) or stimulated with LPS for 3 h. ( e ) ChIP analysis of c-Rel and IRF5 at the promoter of the indicated genes using WT or Traf2 -MKO BMDMs that were either not treated (0) or stimulated for 3 h with LPS. Data are presented as fold relative to the total input DNA and representative of three or more independent experiments. * P <0.05. ( f ) IRF5 and c-Rel were isolated by IP (under denaturing conditions) from whole-cell lysates of DMSO or MG132-treated WT and Traf2 -MKO BMDMs and subjected to IB assays using anti-ubiquitin (top panels) or anti-K48-linked ubiquitin (middle panels) antibodies. Protein lysates were also subjected to direct IB (bottom panels). Data are representative of at least three independent experiments. The error bars represent s.d., and differences between experimental and control groups were determined by Student’s t -test. * P <0.05. Full size image We next analysed the downstream transcription factors known to mediate the proinflammatory TLR signalling. Interestingly, the TRAF2-deficient macrophages had a markedly elevated steady-level of c-Rel and IRF5 ( Fig. 4c ), two major transcription factors mediating proinflammatory cytokine induction [6] , [7] , [8] , [9] , [10] . The TRAF2 deficiency did not affect the expression level of several other transcription factors, including p65 and C/EBPβ ( Fig. 4c ). Consistently, the nuclear level of c-Rel and IRF5, but not C/EBPβ, was drastically higher in the LPS-stimulated TRAF2-deficient macrophages than in the LPS-stimulated WT macrophages ( Fig. 4d ). We found that the nuclear level of p65 was also higher in the TRAF2-deficient macrophages, but this was apparently due to its enhanced nuclear translocation as the cytoplasmic level of p65 was not higher in these mutant cells ( Fig. 4d ). This finding was consistent with the enhanced p65 phosphorylation partially due to aberrant activation of NIK ( Fig. 3a ). To examine the functional significance of c-Rel/IRF5 hyper-activation, we analysed their binding to the promoters of target genes. As expected, ChIP assays revealed binding of c-Rel to the κB enhancer region of two well-defined c-Rel target genes, Il12a and Il12b , on LPS stimulation ( Fig. 4e ). Moreover, this DNA-binding activity of c-Rel was significantly enhanced in the TRAF2-deficient macrophages ( Fig. 4e ). A recent study suggests that IRF5 and canonical NF-κB cooperatively regulate many proinflammatory genes, including Il1b and Il6 , by binding to promoter regions containing the κB enhancer [26] . Consistently, we found that IRF5 bound to the κB region of the Il1 and Il6 genes in LPS-stimulated macrophages, which was greatly enhanced by the TRAF2 deficiency ( Fig. 4e ). Thus, TRAF2 regulates the fate and function of two important proinflammatory transcription factors in macrophages. A previous study suggests that IRF5 expression is induced by M-CSF along with macrophage differentiation [27] . We thus examined whether TRAF2 regulated the expression of IRF5 along with M-CSF-induced macrophage differentiation. We found that the level of both IRF5 and c-Rel was extremely low in bone marrow cells ( Supplementary Fig. 2a ). Consistent with the previous study, M-CSF-induced macrophage differentiation was associated with upregulation of IRF5 ( Supplementary Fig. 2a ). Interestingly, c-Rel was also induced along with the macrophage differentiation ( Supplementary Fig. 2a ). Moreover, the TRAF2 deficiency greatly enhanced the expression of c-Rel and IRF-5 at the level of protein ( Supplementary Fig. 2a ) but not that of mRNA ( Supplementary Fig. 2b ), suggesting a post-translational mechanism of regulation. Indeed, on incubation of macrophages with a proteasome inhibitor, MG132, the level of c-Rel and IRF5 in the Traf2-MKO cells was restored to a level similar to that of the WT cells ( Fig. 4f ). TRAF2 deficiency greatly attenuated the total and K48-linked ubiquitination of c-Rel and IRF5 ( Fig. 4f ). These results suggest that c-Rel and IRF5 actively undergo ubiquitin-dependent degradation in a TRAF2-dependent mechanism. The degradation of c-Rel and IRF5 appeared to occur in the cytoplasm, as they were accumulated in the cytoplasm on incubation of cells with the proteasome inhibitor MG132 ( Supplementary Fig. 2c ). Moreover, c-Rel and IRF5 were also accumulated in the cytoplasm of TRAF2-deficient macrophages and moved to the nucleus only on LPS stimulation ( Fig. 4d ). TRAF3 also negatively regulates c-Rel and IRF5 The TRAF2-mediated c-Rel/IRF5 degradation is remarkably similar to the degradation of NIK [28] , [29] . As the TRAF2-mediated NIK degradation also requires TRAF3, we asked whether TRAF3 might also have a role in mediating degradation of c-Rel and IRF5 in macrophages. We prepared BMDMs from the bone marrow of TRAF3 fl/fl Cre ER or control TRAF3 +/+ Cre ER mice and induced TRAF3 ablation in vitro by culturing the cells in the presence of the Cre ER inducer tamoxifen. Like TRAF2-deficient macrophages, the TRAF3-deficient macrophages did not show obvious alterations in LPS-stimulated activation of p38 or JNK ( Supplementary Fig. 3 ). Interestingly, the TRAF3 ablation resulted in marked accumulation of c-Rel and IRF5 in BMDMs ( Fig. 5a ). The TRAF3 deficiency also enhanced the level of c-Rel and IRF5 along with M-CSF-induced macrophage differentiation ( Fig. 5b ). Consistently, the TRAF3-deficient macrophages displayed hyper-induction of several proinflammatory cytokine genes and inhibited the induction of Il10 gene by both LPS and poly(I:C) ( Fig. 5c and Supplementary Fig. 4b ). 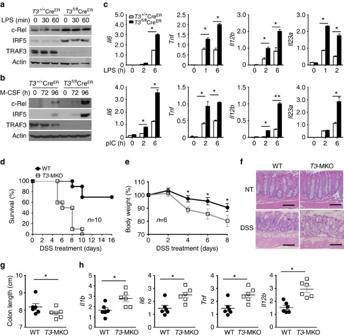Figure 5: TRAF3 controls the fate of c-Rel and IRF5 and negatively regulates inflammation. (a) IB analysis of the indicated proteins in whole-cell lysates of LPS-stimulatedTraf3fl/flCreERor controlTraf3+/+CreERBMDMs differentiated in the presence of the Cre-inducer tamoxifen. (b) IB analysis using whole-cell lysates of M-CSF-treated bone marrow cells from tamoxifen-injectedTraf3fl/flCreERor controlTraf3+/+CreERmice. (c) qRT-PCR analysis of the indicated mRNAs in LPS- or poly(I:C)-stimulatedTraf3+/+CreERandTraf3fl/flCreERBMDMs differentiated in the presence of the Cre-inducer tamoxifen. (d–h)Traf3-MKO and WT control mice were challenged with 3.5% (d) or 3% (E-H) DSS (in drinking water) for 6 days. The mice were monitored for survival (d) and weight loss (e) calculation or killed on day 8 for H&E histology analysis (Scale bar, 100 μm) (f), colon length measuring (g), or flow cytometry analysis of colon macrophages (h). Data are representative of at least three independent experiments. The error bars represent s.d., and differences between experimental and control groups were determined by Student’st-test. For animal survival analysis, the Kaplan–Meier method was adopted to generate graphs, and the survival curves were analysed with log-rank analysis. *P<0.05. Figure 5: TRAF3 controls the fate of c-Rel and IRF5 and negatively regulates inflammation. ( a ) IB analysis of the indicated proteins in whole-cell lysates of LPS-stimulated Traf3 fl/fl Cre ER or control Traf3 +/+ Cre ER BMDMs differentiated in the presence of the Cre-inducer tamoxifen. ( b ) IB analysis using whole-cell lysates of M-CSF-treated bone marrow cells from tamoxifen-injected Traf3 fl/fl Cre ER or control Traf3 +/+ Cre ER mice. ( c ) qRT-PCR analysis of the indicated mRNAs in LPS- or poly(I:C)-stimulated Traf3 +/+ Cre ER and Traf3 fl/fl Cre ER BMDMs differentiated in the presence of the Cre-inducer tamoxifen. ( d – h ) Traf3 -MKO and WT control mice were challenged with 3.5% ( d ) or 3% (E-H) DSS (in drinking water) for 6 days. The mice were monitored for survival ( d ) and weight loss ( e ) calculation or killed on day 8 for H&E histology analysis (Scale bar, 100 μm) ( f ), colon length measuring ( g ), or flow cytometry analysis of colon macrophages ( h ). Data are representative of at least three independent experiments. The error bars represent s.d., and differences between experimental and control groups were determined by Student’s t -test. For animal survival analysis, the Kaplan–Meier method was adopted to generate graphs, and the survival curves were analysed with log-rank analysis. * P <0.05. Full size image Like TRAF2, TRAF3 is upreglated in colonic macrophages ( Fig. 1a ), and TRAF3 upregulation has been associated with human IBD [21] . To examine the role of TRAF3 in the regulation of colonic inflammation, we generated myeloid cell-conditional TRAF3-knockout ( Traf3 -MKO) mice to interrupt its function in innate immune environment. The Traf3 -MKO mice had a normal frequency of macrophages and a slightly higher frequency of neutrophils in the bone marrow ( Supplementary Fig. 4a ). Interestingly, like the Traf2 -MKO mice, the Traf3 -MKO mice had exacerbated colon inflammation in the DSS-induced colitis model, as demonstrated by reduced survival rate, worsened bodyweight loss, as well as more severe mucosal damage and colon shortening ( Fig. 5d–g ). Moreover, colonic macrophages of the DSS-treated TRAF3-deficient mice expressed significantly higher level of proinflammatory cytokines than that of the WT control mice ( Fig. 5h ). Thus, like TRAF2, TRAF3 mediates degradation of c-Rel and IRF5 and functions as an anti-inflammatory factor in innate immune cells. cIAP is involved in degradation of IRF5 and c-Rel Recent studies suggest that TRAF2 and TRAF3 associate with the E3 ubiquitin ligase cIAP1 or cIAP2 to form a complex that mediates the ubiquitination and degradation of NIK [23] , [28] , [29] . It is generally believed that TRAF3 and TRAF2 bind to NIK and cIAP, respectively, and recruit NIK to cIAP through TRAF2-TRAF3 dimerization [28] , [29] . Thus, genetic deficiencies in either TRAF2 or TRAF3 disrupt the cIAP/NIK association and NIK ubiquitination. To date, it has been unknown whether this E3 ubiquitin ligase complex also mediates ubiquitination and degradation of additional substrate proteins. Our finding that ablation of either TRAF2 or TRAF3 in macrophages blocks the ubiquitination and degradation of c-Rel and IRF5 raised the question of whether cIAP is involved in the ubiquitin-dependent degradation of these transcription factors. We tested this possibility using a specific cIAP inhibitor, the Smac mimetic (SM). Interestingly, incubation of the WT macrophages with SM indeed led to accumulation of both c-Rel and IRF5, but had no effect on TRAF2 or TRAF3 ( Fig. 6a ). Moreover, SM had little or no effect on the protein level of c-Rel and IRF5 in the TRAF2-deficient macrophages. Similar results were obtained with the TRAF3-deficient macrophages (data not shown). 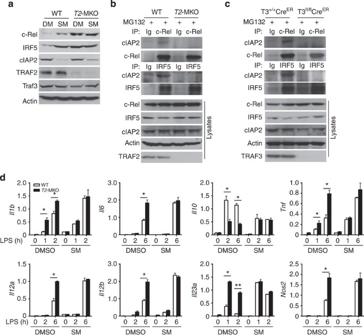Figure 6: cIAP is involved in the regulation of IRF5/c-Rel degradation and proinflammatory cytokine induction. (a) IB analysis of the indicated proteins in the whole-cell lysates of WT andTraf2-MKO BMDMs, treated for 12 h with a Smac mimic (SM) compound or solvent control DMSO (DM). (b,c) BMDMs from WT andTraf2-MKO mice (b) or tamoxifen-treated TRAF3+/+CreERand TRAF3fl/flCreERmice (c) were pretreated with MG132. Whole-cell lysates were subjected to IP using antibodies for IRF5 or c-Rel or a control rabbit IgG (Ig), followed by detecting the precipitated IRF5, c-Rel and their associated cIAP2 by IB. Cell lysates were also subjected to direct IBs (Bottom panels). (d) qRT-PCR analysis of the indicated mRNAs in WT andTraf2-MKO BMDMs, pre-treated for 12 h with a Smac mimic (SM) or DMSO and then stimulated with LPS. Data are mean±s.e.m. of three replicate samples and representative of three independent experiments. The error bars represent s.d., and differences between experimental and control groups were determined by Student’st-test. *P<0.05; **P<0.01. Figure 6: cIAP is involved in the regulation of IRF5/c-Rel degradation and proinflammatory cytokine induction. ( a ) IB analysis of the indicated proteins in the whole-cell lysates of WT and Traf2 -MKO BMDMs, treated for 12 h with a Smac mimic (SM) compound or solvent control DMSO (DM). ( b , c ) BMDMs from WT and Traf2 -MKO mice ( b ) or tamoxifen-treated TRAF3 +/+ Cre ER and TRAF3 fl/fl Cre ER mice ( c ) were pretreated with MG132. Whole-cell lysates were subjected to IP using antibodies for IRF5 or c-Rel or a control rabbit IgG (Ig), followed by detecting the precipitated IRF5, c-Rel and their associated cIAP2 by IB. Cell lysates were also subjected to direct IBs (Bottom panels). ( d ) qRT-PCR analysis of the indicated mRNAs in WT and Traf2 -MKO BMDMs, pre-treated for 12 h with a Smac mimic (SM) or DMSO and then stimulated with LPS. Data are mean±s.e.m. of three replicate samples and representative of three independent experiments. The error bars represent s.d., and differences between experimental and control groups were determined by Student’s t -test. * P <0.05; ** P <0.01. Full size image We next examined the physical association of cIAP with c-Rel or IRF5. We incubated the macrophages with MG132 to equal the level of IRF5 and c-Rel in WT and TRAF2,3-deficient macrophages. Interestingly, co-immunoprecipitation (co-IP) assays readily detected the physical association of cIAP2 with IRF5 and c-Rel in the WT cells, but these molecular interactions were not detected in the TRAF2- and TRAF3-deficient macrophages ( Fig. 6b,c ). These results, along with those described above, suggested that cIAP might target IRF5 and c-Rel in a TRAF2- and TRAF3-dependent manner. To further assess this possibility, we performed co-IP assays to examine whether TRAF2 or TRAF3 could physically interact with IRF5 and c-Rel. When expressed in HEK293 cells, TRAF3, but not TRAF2, strongly interacted with IRF5 and c-Rel ( Supplementary Fig. 5 ). Interestingly, however, co-expression of TRAF2 and TRAF3 allowed TRAF2 to interact with c-Rel and IRF5, suggesting that TRAF3 might serve as the primary interacting protein of c-Rel and IRF5 and recruit these proteins to TRAF2 ( Supplementary Fig. 5 ). To examine the functional involvement of cIAP in proinflammatory cytokine induction, we treated the WT and TRAF2-deficient BMDMs with SM, which is known to induce degradation of cIAP1 and cIAP2 (ref. 30 ). The SM pre-treatment promoted LPS-stimulated expression of a number of proinflammatory cytokines and suppressed Il10 induction in WT BMDMs, but SM had no effect on gene induction in the TRAF2-deficient BMDMs ( Fig. 6d ). This finding was consistent with the requirement of TRAF2 for the association of cIAP with c-Rel and IRF5, thus further suggesting the involvement of the TRAF3-TRAF2-cIAP E3 ubiquitin ligase in the control of proinflammatory TLR signalling in macrophages. TRAF2-deficient macrophages regulate tumour growth in vivo Macrophages are one of the major populations of tumour infiltrating immune cells and play pivotal roles in tumour growth and metastasis [31] . Depending on their polarization phenotypes, macrophages may have anti- or pro-tumour functions. Classically activated (M1) macrophages produce inflammatory cytokines and nitric oxide (NO) that promote anti-tumour immune responses by increasing antigen presentation capacity and inducing the Th1 immunity [32] , [33] , whereas alternatively activated (M2) or M2-like macrophages produce IL-10 and suppress tumour immunity and stimulate tumour progression [34] . As TRAF2 suppresses proinflammatory cytokine induction in macrophages, we surmised that TRAF2 might play a role in regulating the tumour-promoting function of tumour-associated macrophages (TAMs). We examined this hypothesis using a murine melanoma model involving inoculation of B16 melanoma cells into WT or Traf2 -MKO mice. While the B16 tumours grew vigorously in the WT mice, substantially smaller tumours were formed in the Traf2 -MKO mice ( Fig. 7a,b ). The Traf2 -MKO mice also had higher survival rate than the WT mice ( Fig. 7c ). Consistently, the B16 cell-challenged Traf2 -MKO mice had increased frequency of tumour-infiltrating immune (CD45 + ) cells ( Fig. 7d ). Among the CD45 + cells infiltrating into the tumours of Traf2 -MKO mice, there was a considerable increase in the frequency and number of CD4 + and CD8 + effector T cells, whereas the frequency and number of macrophages (CD11b + F4/80 + ) and myeloid-derived suppressor cells (MDSC, CD11b + Gr-1 + ) were either reduced or not altered ( Fig. 7d,e and Supplementary Fig. 6 ). The CD4 + and CD8 + T cells derived from the Traf2 -MKO mouse tumours contained much higher frequency of IFNγ + effector cells than those derived from the WT mouse tumours ( Fig. 7f,g ). These results provided explanation for the stronger tumour rejection ability of the Traf2 -MKO mice. 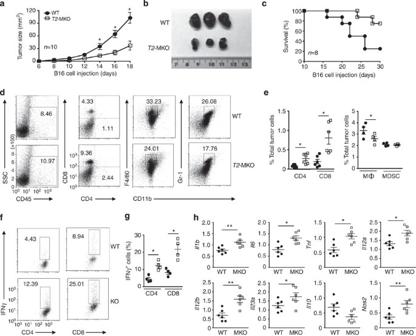Figure 7: TRAF2 functions in myeloid cells to regulate antitumour immunity. WT orTraf2-MKO were injected with 2 × 105(a,bandd–h) or 5 × 105(c) B16 melanoma cells. (a–c) Tumour growth curve (a), a representative picture of day 18 tumours (b), and survival curve (c). (d) Flow cytometric analysis of immune cells (CD45+) infiltrated to day 18 tumours and the frequency of CD4+T cells, CD8+T cells, macrophages (CD11b+F4/80+) and myeloid-derived suppressor cells (MDSCs) (CD11b+Gr-1+) within the CD45+cell population. (e) Summary of flow cytometry data ofdbased on multiple animals, showing the frequency of the indicated cell populations within total tumour cells. (f,g) ICS and flow cytometric analysis of IFNγ+ CD4+and CD8+T cells, presented as a representative plot (f) and a summary graph based on multiple animals with day 18 tumours (g). (h) qRT-PCR analysis of the indicated mRNAs in TAMs derived from day 18 tumours of WT orTraf2-MKO (MKO) mice. Data are mean±s.e.m. value of multiple animals (each circle or square represents a mouse) and representative of three independent experiments. The error bars represent s.d., and differences between experimental and control groups were determined by Student’st-test. *P<0.05; **P<0.01. Figure 7: TRAF2 functions in myeloid cells to regulate antitumour immunity. WT or Traf2 -MKO were injected with 2 × 10 5 ( a , b and d – h ) or 5 × 10 5 ( c ) B16 melanoma cells. ( a – c ) Tumour growth curve ( a ), a representative picture of day 18 tumours ( b ), and survival curve ( c ). ( d ) Flow cytometric analysis of immune cells (CD45 + ) infiltrated to day 18 tumours and the frequency of CD4 + T cells, CD8 + T cells, macrophages (CD11b + F4/80 + ) and myeloid-derived suppressor cells (MDSCs) (CD11b + Gr-1 + ) within the CD45 + cell population. ( e ) Summary of flow cytometry data of d based on multiple animals, showing the frequency of the indicated cell populations within total tumour cells. ( f , g ) ICS and flow cytometric analysis of IFNγ+ CD4 + and CD8 + T cells, presented as a representative plot ( f ) and a summary graph based on multiple animals with day 18 tumours ( g ). ( h ) qRT-PCR analysis of the indicated mRNAs in TAMs derived from day 18 tumours of WT or Traf2 -MKO (MKO) mice. Data are mean±s.e.m. value of multiple animals (each circle or square represents a mouse) and representative of three independent experiments. The error bars represent s.d., and differences between experimental and control groups were determined by Student’s t -test. * P <0.05; ** P <0.01. Full size image To further examine the mechanism by which TRAF2 regulates tumour immunity, we analysed cytokine production in TAMs. The TAMs isolated from tumours of Traf2 -MKO mice expressed higher levels of proinflammatory cytokine genes and Nos2 and lower levels of Il10 ( Fig. 7h ). These data are consistent with those obtained with in vitro macrophage activation experiments ( Fig. 2 ) and suggest that loss of TRAF2 may promote the M1-like anti-tumour function of macrophages. Thus, in addition to regulating colitis, TRAF2 plays a role in macrophage function in tumour microenvironment. The data presented in this paper demonstrated an unexpected mechanism restricting the proinflammatory axis of TLR signalling in macrophages, which involved proteasomal degradation of two major proinflammatory transcription factors, c-Rel and IRF5. This mechanism relied on two TRAF members, TRAF2 and TRAF3, which appeared to function in cooperation with the E3 ubiquitin ligase cIAP to induce ubiquitination of c-Rel and IRF5. Thus, myeloid cell-specific ablation of either TRAF2 or TRAF3 stabilized c-Rel and IRF5 and drastically increased their steady level of expression, rendering macrophages hyper-responsive to TLR ligands and IL-1β in the induction of proinflammatory cytokines. These findings provide a new example for how the ubiquitin-proteasome system regulates TLR signalling and macrophage function. TRAF2 is known as an adaptor molecule mediating signalling from TNFR family members, such as TNFR1 and CD40. Despite the extensive in vitro studies of TRAF2, its in vivo role in the regulation of innate immunity and inflammation has been poorly understood, partly due to the postnatal lethality of the conventional Traf2 -KO mice [35] . In particular, how TRAF2 functions in myeloid cells to regulate TLR signalling and inflammation has not been investigated using in vivo models. Interestingly, upregulated expression of TRAF2, as well as its homologue TRAF3, has been associated with human IBD [19] , [20] , [21] . We also detected a considerably higher level of TRAF2 and TRAF3 in colon macrophages, compared with the spleen and peritoneal macrophages, of colitis-induced mice. Our data revealed that TRAF2, as well as TRAF3, negatively regulated inflammation in DSS-induced colitis, thus suggesting the involvement of these factors in a negative-feedback mechanism that restricts inflammation. A previous study suggests that TRAF2 prevents spontaneous colitis by mediating the survival of colonic epithelial cells [36] . While this function is consistent with the positive role of TRAF2 in mediating TNF receptor-induced survival signals in epithelial cells, our current study demonstrated a novel anti-inflammatory function of TRAF2 involving negative regulation of TLR signalling in myeloid cells. In addition to regulating inflammation, TRAF2 had a role in modulating tumour immunity. Myeloid cell-specific deletion of TRAF2 greatly enhanced the frequency of tumour-infiltrating T cells, particularly CD8 T cells, and promoted tumour rejection. TRAF2-deficient TAMs produced elevated levels of proinflammatory cytokines and iNOS, suggesting an M1-like phenotype that is known to promote anti-tumour T-cell responses [34] . In the TNFR pathways, TRAF2 serves as a positive signalling mediator for the activation of IKK and JNK and their downstream transcription factors, NF-κB and AP1, respectively [37] , [38] . We found that TRAF2 deficiency in macrophages had no effect on LPS-stimulated JNK activation and only partially inhibited IKK activation. Interestingly, despite the moderately weakened IKK activation, the TRAF2-deficient macrophages were hyper-responsive to LPS for proinflammatory cytokine induction. Our data suggest that TRAF2 negatively regulates the proinflammatory axis of TLR signalling by mediating degradation of c-Rel and IRF5, key transcription factors for proinflammatory cytokine gene induction. Consistent with previous reports [39] , [40] , [41] , we found that TRAF3 also negatively regulated LPS-stimulated proinflammatory cytokine production. It has been proposed that TRAF3 may inhibit the activation of JNK and p38 through regulating the cytoplasmic translocation of the MyD88 signalling complex [15] . However, TRAF3 knockout or knockdown does not substantially elevate LPS-stimulated phosphorylation of JNK or p38 (refs 39 , 40 , 41 ). Using BMDMs derived from both Traf3 -MKO and the inducible Traf3 fl/fl Cre ER mice, we further demonstrated that TRAF3 deficiency had no major effect on p38/JNK activation. Furthermore, the role of TRAF3 in TLR regulation was not limited to the MyD88 pathway, as TRAF3 deficiency also promoted proinflammatory gene induction by the TRIF-dependent TLR ligand poly(I:C). Our data suggest that TRAF3, like TRAF2, functions to mediate degradation of c-Rel and IRF5. TRAF2 and TRAF3 are known to form a complex with the E3 ubiquitin ligase cIAP (cIAP1 or cIAP2) that mediates degradation of NIK [28] , [29] . To date, it has been thought that this E3 complex specifically mediates degradation of NIK. Our current study revealed that all three components of this E3 complex were required for c-Rel/IRF5 degradation in macrophages, suggesting that the TRAF3-TRAF2-cIAP complex may also function as an E3 of c-Rel and IRF5 ( Supplementary Fig. 7 ). Our findings are consistent with the recent reports that the cIAP antagonist SM has proinflammatory actions in myeloid cells and macrophages [42] , [43] . We further showed that SM greatly promoted LPS-stimulated expression of proinflammatory cytokines in BMDMs. Our findings shed new light on the in vivo proinflammatory and immunostimulatory roles of SM. Our data suggested that the deregulated NIK activation in TRAF2-deficient macrophages only played a minor role in mediating the hyper-induction of proinflammatory cytokines by LPS, further emphasizing the role of IRF5 and c-Rel in this proinflammatory action. However, the deregulated NIK activation did cause some level of activation of the canonical NF-κB signalling, as suggested by the enhanced phosphorylation and nuclear translocation of p65. Our recent study demonstrates that the NIK-induced noncanonical NF-κB pathway negatively regulates the induction of type I interferons [44] . Hence, it is likely that the TRAF3-TRAF2-cIAP complex may regulate both NIK-dependent and IRF5/c-Rel-dependent signalling events involved in the induction of proinflammatory cytokines and type I interferons ( Supplementary Fig. 7 ). Mice Traf2 -flox and Traf3 -flox mice were provided by Dr Robert Brink (Garvan Institute of Medical Research) [45] . These mice were crossed with lysozyme 2-Cre ( Lyz2 -Cre) mice (Jackson Lab) [46] to produce age-matched Traf2 fl/fl lyz2 Cre/+ (termed Traf2 -MKO) and Traf2 fl/fl - lyz 2 +/+ (termed WT) mice or Traf3 fl/fl lyz2 Cre/+ (termed Traf3 -MKO) and Traf3 fl/fl - lyz2 +/+ (termed WT) mice. The NIK-KO mice were provided by Amgen [47] . In some experiments, Traf2 -MKO mice were further crossed with NIK-KO mice for generating double-KO mice. The NIK-KO mice had a 129SvEv background, and all other mouse strains had a B6;129 mixed background. The mice were maintained in specific pathogen-free facility of The University of Texas MD Anderson Cancer Center, and all animal experiments were conducted in accordance with protocols approved by the Institutional Animal Care and Use Committee. Antibodies and reagents Antibodies for RelB (C-19, 1:1,000), Lamin B (C-20, 1:1,000), NIK (H248, 1:1,000), TRAF2 (C-20, 1:1,000), TRAF3 (H-122, 1:1,000), cIAP2 (H85, 1:1,000), ERK (K-23, 1:5,000), phospho-ERK (E-4, 1:3,000), JNK1 (C-17, 1:1,000), p38 (H-147, 1:1,000), phospho-p65 (Ser529, 1:1,000), IKKα (H744, 1:1,000), IKKβ (H-4, 1:1,000), IKKγ (FL-419, 1:1,000), ubiquitin (P4D1, 1:1,000) and c-Rel (sc71, 1:3,000), as well as a control rabbit IgG (sc-2027, 1:1,000), were from Santa Cruz Biotechnology. Antibodies for phosho-TAK1 (Thr187, 1:1,000), phospho-IκBα (Ser32, 1:1,000), phospho-JNK (Thr180/Tyr185, 1:1,000), phospho-p38 (Thr180/Tyr182, 1:1,000) and IRF5 (4950S, 1:1,000) were purchased from Cell Signaling Technology. Anti-Actin (C-4, 1:10,000) was from Sigma, and anti-TAK1 (1:1,000) was provided by Dr Jun Ninomiya-Tsuji (North Carolina State University). Antibody for p100/p52 (TB4, 1:8,000) was from National Cancer Institute Preclinical Repository. Other antibodies were described previously [48] . Fluorescence-labelled antibodies are listed in the section of flow cytometry and cell sorting. LPS (derived from Escherichia coli strain 0127:B8) and CpG (2216) were from Sigma-Aldrich. Poly (I:C) was from Amersham, dextran sulfate sodium salt (DSS) was from MP Biomedicals, and recombinant murine M-CSF and IL-1β were from Peprotech. Smac mimic was kindly provided by Dr Xiaodong Wang (National Institute of Biological Sciences, Beijing). Flow cytometry, cell sorting and intracellular cytokine staining (ICS) Single-cell suspensions of colon tissue, B16 melanoma, or bone marrow were subjected to flow cytometry using FACSAria (BD Bioscience) and the following.fluorescence-labelled antibodies from eBioscience: PB-conjugated anti-IFNγ, anti-CD4 and anti-CD11c; PE-conjugated anti-F4/80 and anti-CD45; PerCP5.5-conjugated anti-Gr-1 (Ly6G) and anti-CD45; APC-conjugated anti-CD11b; and APC-CY7-conjugated anti-CD8. The macrophages in colon tissue and B16 melanoma were stained with APC-conjugated anti-CD11b and PE-conjugated anti-F4/80 and sorted by flow cytometry using FACSAriaII (BD Bioscience). For ICS, the tumour-infiltrating T cells were stimulated for 4 h with PMA plus ionomycin in the presence of monensin and then subjected to intracellular IFN-γ staining and flow cytometry. ELISA and Real-time quantitative RT-PCR (qRT-PCR) Supernatants of in vitro cell cultures were analysed by ELISA using a commercial assay system (eBioScience). For qRT-PCR, total RNA was isolated using TRI reagent (Molecular Research Center) and subjected to cDNA synthesis using RNase H-reverse transcriptase (Invitrogen) and oligo (dT) primers. qRT-PCR was performed in triplicates, using iCycler Sequence Detection System (Bio-Rad) and iQTM SYBR Green Supermix (Bio-Rad). The expression of individual genes was calculated by a standard curve method and normalized to the expression of Actb . The gene-specific PCR primers (all for mouse genes) are shown in Supplementary Table 1 . Immunoblot (IB), IP and kinase assays Whole-cell lysates or subcellular extracts were prepared and subjected to IB and IP assays as described [49] . The samples were resolved by 8.25% SDS–PAGE. After electrophoresis, separated proteins were transferred onto polyvinylidene difluoride membrane (Millipore). For IB assays, the polyvinylidene difluoride membrane was blocked with 5% non-fat milk. After incubation with a specific primary antibody, horseradish peroxidase-conjugated secondary antibody was applied. The positive immune reactive signal was detected by ECL (Amersham Biosciences). For kinase assays, the IKK complex was isolated from WT and Traf2 -MKO BMDMs by IP (using anti-IKKγ) and subjected to IKK kinase assay (KA) using GST-IκBα (1–54) (1 μg) as a substrate as previously described [50] . Full-size images are presented in Supplementary Figs 8–11 . Ubiquitination assays Cells were pretreated with MG132 for 2 h and then lysed with a Nonidet P-40 lysis buffer (50 mM Tris–HCl, pH7.5, 120 mM NaCl, 1% Nonidet P-40, 1 mM EDTA, 1 mM DTT) containing 6 M urea and protease inhibitors. c-Rel and IRF5 were isolated by IP with antibodies for c-Rel (sc-71) and IRF5 (4950S), respectively, and the ubiquitinated c-Rel or IRF5 was detected by IB using an anti-ubiquitin (P4D1). For transfection models, expression vectors encoding c-Rel or HA-IRF5 was transfected into HEK293 cells along with HA-ubiquitin and other indicated vectors. The cells were pretreated with MG132 for 2 h and then lysed for IP followed by detecting ubiquitination by IB using anti-ubiquitin. Chromatin immunoprecipitation (ChIP) assays BMDMs (6 × 10 7 ) were stimulated for 3 h with LPS, fixed in 1% formaldehyde and then sonicated as previously described [51] . Lysates (from 2 × 10 7 cells in 3 ml) were subjected to IP with the indicated antibodies, and the precipitated DNA was then purified by Qiaquick columns (Qiagen) and quantified by QPCR using primers listed in Supplementary Table 1 to amplify NF-κB-binding region of the different gene promoters. The precipitated DNA is presented as percentage of the total input DNA ( y -axis). DSS-induced colitis For lethality analysis, mice were supplied with 3.5% DSS in drinking water (MP Biomedicals) for 6 days and replaced with normal drinking water for the rest of experimental time. The treated mice were monitored every other day, and moribund mice were killed based on protocols approved by the IACUC of the University of Texas MD Anderson Cancer Center. For inflammation studies, mice were treated with a lower dose (3%) of DSS to prevent early lethality. Body weight was measured every other day for up to 8 days, and the mice were then killed for measuring colon length, histology analysis and immune cell isolation from the mucosa. For isolating colon macrophages, the colon was cut and digested with 0.25 mg ml −1 collagenase A (Sigma-Aldrich) and 25 U ml −1 DNase (Roche Diagnostics, Indianapolis, IN) for 20 min at 37 °C. Cells were harvested by passing the suspension through a cell strainer (BD Biosciences, San Diego, CA), followed by centrifugation. Colonic macrophages were isolated from colonic cells by FACS sorting using CD11b and F4/80 markers (double positive). Inflammation cytokine gene expression was analysed by qRT-PCR. Macrophage preparation and stimulation BMDMs were prepared essentially as previously described [48] . In brief, bone marrows were isolated from the femurs of young adult mice and cultured for 5 days in a DMEM medium supplemented with M-CSF conditional medium. For inducible ablation of TRAF3 in BMDMs, the bone marrows of Traf3 +/+ Cre ER or Traf3 fl/fl Cre ER mice were differentiated in the M-CSF medium in the presence of tamoxifen (1 μg ml −1 ). For inducible ablation of TRAF3 in bone marrow cells, the Traf3 +/+ Cre ER and Traf3 fl/fl Cre ER mice were injected i.p with tamoxifen (5 mg per mouse) every other day for three times and killed after 7 days for bone marrow cell preparation. For peritoneal macrophage isolation, WT and Traf2 -MKO mice were killed, and the peritoneal cavity was lavaged with 8 ml of RPMI 1640 medium. The medium recovered from three mice was pooled, and cells were collected by centrifugation and plated onto 12-well plates in a density of 1 × 10 6 cells ml −1 . Macrophages were allowed to adhere for 2 h (37 °C, 5% CO2), washed with fresh medium to remove unattached cells and incubated overnight. BMDMs and peritoneal macrophages were starved overnight in medium supplemented with 0.5% FCS before being stimulated with LPS (1 μg ml −1 for IB experiments and 100 ng ml −1 for cytokine induction experiments), poly(I:C) (20 μg ml −1 ), CpG (2216, 5 μM) and murine recombinant IL-1β (20 ng ml −1 ). Total and subcellular extracts were prepared for IB assays, and total RNA was prepared for qRT-PCR assays. The B16-infiltrating macrophages were isolated by FACS sorting with CD11b and F4/80 marker (double positive) and used for qRT-PCR and IB assays. B16 model of melanoma WT and Traf2 -MKO mice were injected s.c. with 5 × 10 5 B16 melanoma cells. The injected mice were monitored for tumour growth every other day, and lethality was defined when mice had a tumour size reaching 225 mm 2 based on protocols approved by the IACUC of University of Texas MD Anderson Cancer Center. For analyses of tumour growth rate and tumour-infiltrating immune cells, a lower number (2 × 10 5 ) of B16 cells were injected to prevent lethality during the course of the experiment. To minimize individual variations, littermate WT and Traf2 -MKO mice were used. Mice were randomly selected for tumour injection, and analysis of tumour size was done in a blinded manner. To analyse tumour-infiltrating immune cells, tumour tissues were treated with 0.25 mg ml −1 collagenase A (Sigma-Aldrich) and 25 U ml −1 DNase (Roche Diagnostics, Indianapolis, IN) for 20 min at 37 °C, and the cells were passed through a plastic mesh. The resulting dissociated cells were collected by centrifugation, resuspended in Red Blood Cell Lysis Buffer for 3 min and washed twice in PBS. The cells were subjected to flow cytometry analysis, and TAMs were isolated by cell sorting based on CD11b + F4/80 + surface markers. Statistical analysis Prism software was used for two-tailed unpaired t -tests. P values<0.05 and 0.01 are considered significant and very significant, respectively. How to cite this article : Jin, J. et al . Proinflammatory TLR signalling is regulated by a TRAF2-dependent proteolysis mechanism in macrophages. Nat. Commun. 6:5930 doi: 10.1038/ncomms6930 (2015).